ArabidopsisFLC clade members form flowering-repressor complexes coordinating responses to endogenous and environmental cues The developmental transition to flowering is timed by endogenous and environmental signals through multiple genetic pathways. In Arabidopsis , the MADS-domain protein FLOWERING LOCUS C is a potent flowering repressor. Here, we report that the FLOWERING LOCUS C clade member MADS AFFECTING FLOWERING3 acts redundantly with another clade member to directly repress expression of the florigen FLOWERING LOCUS T and inhibit flowering. FLOWERING LOCUS C clade members act in partial redundancy in floral repression and mediate flowering responses to temperature, in addition to their participation in the flowering-time regulation by vernalization and photoperiod. We show that FLOWERING LOCUS C, MADS AFFECTING FLOWERING3 and three other clade members can directly interact with each other and form nuclear complexes, and that FLOWERING LOCUS C- dependent floral repression requires other clade members. Our results collectively suggest that the FLOWERING LOCUS C clade members act as part of several MADS-domain complexes with partial redundancy, which integrate responses to endogenous and environmental cues to control flowering. When to flower is a critical developmental switch for reproductive success in plant life cycle. In Arabidopsis thaliana , a facultative long-day plant, the transition to flowering is timed by endogenous and environmental signals. Multiple genetic pathways such as the photoperiod, vernalization, thermosensory and aging pathways responding, respectively, to day-length change, prolonged cold exposure, ambient temperature fluctuation and plant age, form an integrated regulatory network to control the timing of flower initiation under a given environment [1] , [2] . In the Arabidopsis flowering-regulatory network, the MADS-domain transcription factor FLOWERING LOCUS C (FLC) functions as a potent floral repressor [3] , [4] . FRIGIDA ( FRI ) activates FLC expression to confer a winter-annual growth habit (late flowering if without vernalization) [5] , [6] . Vernalization, exposure to a typical cold winter, represses FLC expression enabling plants to flower next spring [7] , [8] , [9] , [10] . In the rapid-cycling accessions lack of a functional FRI , FLC expression is repressed by ‘autonomous-pathway’ genes such as FCA , FPA , FLD and LUMINIDEPENDENS [1] , [7] , [11] . The FLC protein associates with another MADS-box domain protein SHORT VEGETATIVE PHASE (SVP) to directly repress the expression of the conserved florigen FLOWERING LOCUS T ( FT ) and another flowering promoter SUPPRESSOR OF OVEREXPRESSION OF CO 1 ( SOC1 ), resulting in floral repression [12] , [13] , [14] , [15] . Besides FLC , there are five FLC homologues in Arabidopsis genome, including FLOWERING LOCUS M ( FLM ) /MADS AFFECTING FLOWERING 1, and MAF2-MAF5 that are arranged in tandem as a 22-kb cluster [16] , [17] , [18] . Like FLC , FLM represses flowering [17] , [18] ; in addition, FLM appears to act partly in the photoperiod pathway and partly in the thermosensory pathway to regulate flowering time [19] , [20] . Furthermore, MAF2 also acts as a floral repressor and loss of MAF2 function leads to accelerated flowering upon vernalization [16] . Another FLC clade member, MAF4 represses flowering as well [21] . MAF5 is normally repressed and its ectopic overexpression under non-inductive short days causes late-flowering [22] . To date, the biological function of MADS AFFECTING FLOWERING3 ( MAF3 ) remains elusive. FT and FT homologues in other plants constitute a major component of florigen (flowering ‘hormone’ or inducer) [2] , [23] . FT has a central role in flowering promotion and functions as a floral pathway integrator, and multiple pathways converge at FT to regulate flowering time [2] , [23] . The photoperiod pathway acts through CONSTANS ( CO ) whose expression is controlled by the circadian clock, to activate FT expression in leaf veins specifically at the end of inductive long days [2] , [24] . The FT protein is transported from leaf (phloem companion cells) to the shoot apical meristem to induce flowering [25] , [26] , [27] , [28] . FT expression is regulated by ambient temperature as well, and the thermosensory pathway acts mainly through FT , independently of the photoperiod pathway, to regulate flowering time [20] , [29] . Under cool conditions (for example, 16 °C), decreased FT expression causes a flowering delay [15] , whereas growth temperature rises (for example, 17 to 27 °C) upregulate the expression of bHLH transcription factor PHYTOCHROME INTERACTING FACTOR 4 ( PIF4 ) that directly activates FT expression to promote flowering [30] . Some MADS-domain transcription factors function as part of a complex to regulate gene expression, and recent studies have revealed that MIKC c -type MADS-domain proteins can assemble into quaternary complexes [31] , [32] . The MADS domain typically recognizes and binds to CArG motifs, and MADS-domain complexes consisting of two dimers may bind to a target gene typically with two CArG motifs [31] , [32] . Several MADS-domain ‘floral quartet’ complexes involved in floral organ development have been described [31] , [32] . The FLC clade members are MIKC c -type proteins; FLC has been shown to directly associate with another MIKC c -type protein SVP and both proteins recognize CArG motifs in SOC1 , and presumably FT , to repress their expression [12] . However, whether FLC and FLC clade members form complexes to control the floral transition is essentially unknown. In this study, we show that MAF3 acts redundantly with FLM to directly repress the expression of conserved florigen FT and inhibits flowering, and that FLM also overlaps with FLC , MAF2 and MAF4 in floral repression. Furthermore, we found that FLC, FLM and MAF2-MAF4 proteins directly interact with each other and form nuclear complexes, and that FLC -dependent flowering repression requires other FLC clade members. In addition, we uncovered that FLM binding to FT chromatin is partly dependent on other FLC clade members. Our results collectively suggest that the FLC clade members together with SVP form MADS-domain complexes to regulate flowering time in response to endogenous factors and environmental cues. MAF3 is a floral repressor To elucidate MAF3 function, we identified two T-DNA insertion mutants maf3–1 and maf3–2 ( Supplementary Fig. S1a ). In both mutants, the full-length transcription of MAF3 was completely disrupted ( Supplementary Fig. S1c ). Grown in long days (LDs, 16-h light/8-h dark), maf3-1 and maf3-2 flowered slightly earlier than wild-type Col (WT), whereas flc maf3-2 and flm maf3-2 flowered apparently earlier than flc and flm , respectively, ( Fig. 1a ); in addition, both flc flm maf3-1 and flc flm maf3-2 flowered substantially early and earlier than flc flm ( Fig. 1a , Supplementary Fig. S1b ). In short days, the maf3 mutation strongly enhanced the early-flowering phenotype of flm ( Fig. 1b ), indicating a functional redundancy of MAF3 with FLM in Arabidopsis floral repression. 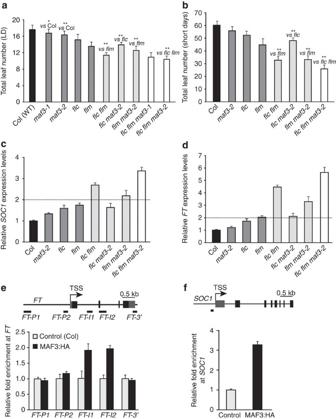Figure 1:MAF3is a floral repressor and repressesFTandSOC1expression. (a) Flowering times of the indicated genotypes grown in LDs (at 22 °C). Total number of primary leaves formed before flowering was scored for each line (17–22 plants per line). Asterisks indicate statistically significant differences in the means between the indicated genotypes, as revealed by two-tailed Student’st-test (*P<0.05; **P<0.01). Bars indicate s.d. (b) Flowering times of the indicated genotypes grown in short days. Ten to twelve plants were scored for each line. (c,d) RelativeSOC1(c) andFT(d) expression levels in the seedlings of indicated genotypes grown in LDs. TheSOC1orFTtranscript levels in each line harvested at ZT12 (12 h after dawn) were quantified by qRT–PCR, and normalized to the endogenous controls includingUBIQUITIN10(UBQ10) andTUBULIN2(TUB2); relative expression to Col (WT) is presented. Bars indicate s.d. of six measurements (three for each control). Biological repeats of these analyses are presented asSupplementary Fig. S2a,b. (e–f) ChIP analysis of MAF3:HA enrichment at theFTandSOC1loci at the end of LD (ZT16). The amounts of immunoprecipitated genomic DNA were measured by qPCR, and normalized to the endogenous controlTUBULIN8(TUB8). The fold enrichments of MAF3:HA protein in each examined region ofFTandSOC1in theMAF3:HAline over Col (control) are shown. Error bars indicate s.d. of three measurements. A biological repeat of this analysis is shown inSupplementary Fig. S4b,c. Figure 1: MAF3 is a floral repressor and represses FT and SOC1 expression. ( a ) Flowering times of the indicated genotypes grown in LDs (at 22 °C). Total number of primary leaves formed before flowering was scored for each line (17–22 plants per line). Asterisks indicate statistically significant differences in the means between the indicated genotypes, as revealed by two-tailed Student’s t -test (* P <0.05; ** P <0.01). Bars indicate s.d. ( b ) Flowering times of the indicated genotypes grown in short days. Ten to twelve plants were scored for each line. ( c , d ) Relative SOC1 ( c ) and FT ( d ) expression levels in the seedlings of indicated genotypes grown in LDs. The SOC1 or FT transcript levels in each line harvested at ZT12 (12 h after dawn) were quantified by qRT–PCR, and normalized to the endogenous controls including UBIQUITIN10 ( UBQ10 ) and TUBULIN2 ( TUB2 ); relative expression to Col (WT) is presented. Bars indicate s.d. of six measurements (three for each control). Biological repeats of these analyses are presented as Supplementary Fig. S2a,b . ( e – f ) ChIP analysis of MAF3:HA enrichment at the FT and SOC1 loci at the end of LD (ZT16). The amounts of immunoprecipitated genomic DNA were measured by qPCR, and normalized to the endogenous control TUBULIN8 ( TUB8 ). The fold enrichments of MAF3:HA protein in each examined region of FT and SOC1 in the MAF3:HA line over Col (control) are shown. Error bars indicate s.d. of three measurements. A biological repeat of this analysis is shown in Supplementary Fig. S4b,c . Full size image FLC directly represses the expression of FT and SOC1 to repress flowering. This prompted us to measure FT and SOC1 expression changes upon functional loss of MAF3 , FLM and/or FLC . SOC1 transcript levels were increased slightly in flm and flc mutants, but strongly in the flc flm double mutant relative to WT; loss of MAF3 function had little effect on SOC1 expression, whereas upon combined functional loss of MAF3 with FLM , the SOC1 transcript levels were apparently increased ( Fig. 1c ). With regard to FT expression, it was moderately increased in flc or flm , but slightly in maf3 relative to WT; the combined functional loss of MAF3 with FLM led to a synergistic increase of FT transcript levels (about threefold relative to WT), and a substantial increase (about fourfold) was observed upon combined loss of FLM with FLC function, which was strongly enhanced by further loss of MAF3 function (about sixfold in flc flm maf3 relative to WT) ( Fig. 1d ; Supplementary Fig. S2 ). These results show that FLM overlaps with MAF3 and FLC to repress FT expression. It is well known that FT, the mobile florigen, moves from leaf to the shoot apex where it forms a complex with FD to induce flowering [33] , [34] . We further examined FD expression in Col, maf3 flc , maf3 flm and maf3 flc flm seedlings and found that it was slightly increased in the mutants relative to WT ( Supplementary Fig. S3 ). In short, we found that FLM overlaps with MAF3 and FLC to repress FT and SOC1 expression, and that these three genes have a great role in FT repression, leading to floral repression. MAF3 binds to FT and SOC1 chromatin Next, we examined whether the MAF3 protein could directly interact with the FT and SOC1 loci, using a transgenic line (homozygous T 3 and in the maf3–2 background) expressing a fully-functional MAF3:HA driven by its native promoter ( Supplementary Fig. S4a ). We conducted chromatin immunoprecipitation (ChIP) assays using MAF3:HA seedlings grown in LDs, and found that MAF3:HA, like FLC [13] , [14] , was enriched in the first and second introns, but not in 5′ promoter or 3′ end of FT , and bound to the proximal promoter of SOC1 at the examined time point ZT16 (ZT for Zeitgeber time, hours after dawn) ( Fig. 1e , Supplementary Fig. 4b,c ). Thus, MAF3 directly interacts with the FT and SOC1 loci to repress their expression. MAF3 and its repression of FT expression exhibit a diurnal change Day length or day/night cycle regulates flowering time via the photoperiod pathway [24] , we sought to address whether day/night cycles could affect MAF3 protein accumulation. The levels of MAF3:HA protein in the functional MAF3:HA -expressing line were measured every 4 h under the 24-h LD cycle. MAF3 protein accumulation displayed a diurnal change, and peaked at ZT4 and ZT16 ( Fig. 2a ). FT expression is controlled by the circadian clock through CO and peaks at the end of LDs [24] . Next, we examined at what time MAF3 represses FT expression by measuring FT transcript levels in WT, maf3 , flm and maf3 flm seedlings in LDs. Upon the combined loss of MAF3 and FLM function, FT transcript levels were greatly increased at the day’s end (ZT16) ( Fig. 2c , Supplementary Fig. S5a,b ), consistent with MAF3 protein accumulation and binding to FT chromatin at this time ( Fig. 1e , Fig. 2a ). Interestingly, at ZT4 FT expression was only slightly de-repressed in flm maf3 ( Fig. 2c ), indicating that other factors may repress FT expression at this time in the absence of FLM and MAF3 . Taken together, our results show that MAF3 protein accumulates and has a great role in the repression of FT expression at the end of LDs. 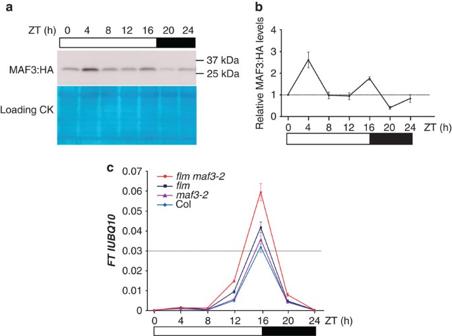Figure 2: MAF3 protein exhibits a diurnal change and repressesFTexpression at the late day in LDs. (a) MAF3:HA protein levels in Col seedlings over a 24-h LD cycle, examined by western blotting. Total proteins from the blotting membrane stained with Amido Black serve as loading controls; white and dark bars for light and dark periods, respectively. (b) Relative MAF3:HA protein levels over a 24-h LD cycle. Band intensities of triplicate technical repeats were quantified by the ImageJ 1.44j program, and relative levels to ZT0 are presented. Note that the time of the day has a significant effect on the MAF3 protein levels in the seedlings, as revealed by a single-factor ANOVA test (P<0.01). (c)FTmRNA levels in the seedlings of indicated lines grown on half-MS media over a 24-h LD cycle. TheFTlevels were quantified by qRT–PCR, normalized toUBQ10, and calculated as 2−ΔCt(ΔCt=Ct(FT)−Ct(UBQ10)). Bars indicate s.d. of triplicate measurements. RelativeFTlevels normalized to another reference geneTUB2are shown inSupplementary Fig. S5a. A biological repeat of this analysis is presented asSupplementary Fig. S5b. Figure 2: MAF3 protein exhibits a diurnal change and represses FT expression at the late day in LDs. ( a ) MAF3:HA protein levels in Col seedlings over a 24-h LD cycle, examined by western blotting. Total proteins from the blotting membrane stained with Amido Black serve as loading controls; white and dark bars for light and dark periods, respectively. ( b ) Relative MAF3:HA protein levels over a 24-h LD cycle. Band intensities of triplicate technical repeats were quantified by the ImageJ 1.44j program, and relative levels to ZT0 are presented. Note that the time of the day has a significant effect on the MAF3 protein levels in the seedlings, as revealed by a single-factor ANOVA test ( P <0.01). ( c ) FT mRNA levels in the seedlings of indicated lines grown on half-MS media over a 24-h LD cycle. The FT levels were quantified by qRT–PCR, normalized to UBQ10 , and calculated as 2 −ΔCt (ΔC t =C t ( FT )−C t ( UBQ10 )). Bars indicate s.d. of triplicate measurements. Relative FT levels normalized to another reference gene TUB2 are shown in Supplementary Fig. S5a . A biological repeat of this analysis is presented as Supplementary Fig. S5b . Full size image MAF2 and MAF4 overlap with FLM to repress FT expression and flowering MAF2 and MAF4, like MAF3, are closer to FLM than to FLC ( Supplementary Fig. S6 ); hence, we further examined genetic interactions of flm with maf2 and maf4 . Under LDs, the flm maf2 double mutant flowered much earlier than either single mutants ( Fig. 3a ). In addition, we found that the maf4 mutation enhanced moderately the early-flowering phenotype of flm in LDs ( Fig. 3a ), whereas under short days, flm maf4 flowered substantially earlier than flm ( Supplementary Fig. S7a ). Furthermore, we checked whether there is any genetic interaction of FLM with MAF5 . Loss of MAF5 function did not affect flowering in either WT or the flm flc background ( Supplementary Fig. S7b ), indicating that MAF5 has a limited role in flowering-time regulation. 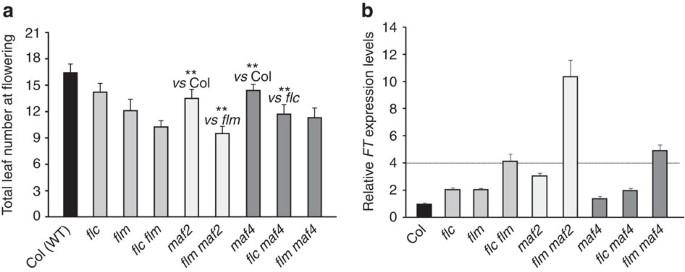Figure 3:FLMoverlaps with otherFLCclade members to repressFTexpression. (a) Flowering times of the indicated genotypes grown in LDs (at 22 °C). Ten to nineteen plants for each line were scored. Double asterisks indicate statistically significant differences (P<0.01), revealed by two-tailed Student’st-test, in the means between the indicated genotypes. Bars indicate s.d. (b) RelativeFTexpression levels in the seedlings of indicated genotypes at ZT12 in LDs, as quantified by qRT–PCR. TheFTlevels were normalized toUBQ10andTUB2; bars indicate s.d. of six measurements (three for each control). A biological repeat of this analysis is presented asSupplementary Fig. S5c. Figure 3: FLM overlaps with other FLC clade members to repress FT expression. ( a ) Flowering times of the indicated genotypes grown in LDs (at 22 °C). Ten to nineteen plants for each line were scored. Double asterisks indicate statistically significant differences ( P <0.01), revealed by two-tailed Student’s t -test, in the means between the indicated genotypes. Bars indicate s.d. ( b ) Relative FT expression levels in the seedlings of indicated genotypes at ZT12 in LDs, as quantified by qRT–PCR. The FT levels were normalized to UBQ10 and TUB2 ; bars indicate s.d. of six measurements (three for each control). A biological repeat of this analysis is presented as Supplementary Fig. S5c . Full size image Next, we examined FT expression in seedlings upon functional loss of FLM , MAF2 and/or MAF4 . FT transcript levels were greatly increased in maf2 flm and maf4 flm relative to respective single mutants under LDs: the maf2 flm double with about tenfold increase relative to WT (only a moderate increase in maf2 or flm ) and fivefold increase for maf4 flm (only a slight increase in maf4 ) ( Fig. 3b ), suggesting synergistic interactions of flm with maf2 and maf4 . Together, these observations show that FLM overlaps with MAF2 and MAF4 to repress FT expression. FLC clade members are required for flowering delay by temperature drop The thermosensory pathway acts largely through FT to regulate flowering time in response to growth temperature fluctuations; recent studies reveal that FLM and SVP may act in this pathway [15] , [20] . We asked whether other members of the FLC clade could be involved in thermo-regulation of flowering. Owing to functional redundancy of FLM with FLC , MAF2 and MAF4 , we created flm flc maf2 and flm flc maf4 triple mutants and measured flowering-delay responses of single and triple mutants of the FLC clade members upon a growth temperature drop from 23 to 16 °C. In WT, the temperature drop caused a more than onefold delay of flowering time, whereas the FLC clade mutants, including flc , flm , maf2 , maf3 and maf4 were less sensitive to the drop compared with WT, among which flm displayed the least sensitivity ( Fig. 4a–b , Supplementary Fig. S8 ). These data show that the thermo responses of flowering in these FLC clade mutants are partially disrupted; hence, these genes are all partly required for the temperature drop-induced flowering delay. 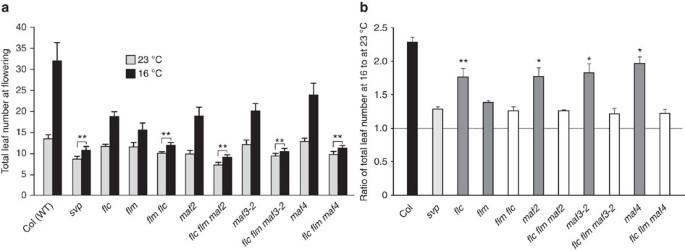Figure 4: Effect of growth temperature on flowering times of theFLCclade mutants. (a) Flowering times of the indicated genotypes grown at 16 and 23 °C (in LDs). Thirteen to twenty-three plants for each line were scored; bars for s.d. One of the two additional biological repeats is presented inSupplementary Fig. S8. (b) Flowering sensitivity of theFLCclade mutants to the temperature drop, indicated by the ratio of total leaf number at 16 °C to that at 23 °C. The values are the averages of three biological repeats; bars for s.d. An asterisk indicates a statistically significant difference in the means between Col and an indicated genotype, as revealed by two-tailed Student’st-test (*P<0.05; **P<0.01). Figure 4: Effect of growth temperature on flowering times of the FLC clade mutants. ( a ) Flowering times of the indicated genotypes grown at 16 and 23 °C (in LDs). Thirteen to twenty-three plants for each line were scored; bars for s.d. One of the two additional biological repeats is presented in Supplementary Fig. S8 . ( b ) Flowering sensitivity of the FLC clade mutants to the temperature drop, indicated by the ratio of total leaf number at 16 °C to that at 23 °C. The values are the averages of three biological repeats; bars for s.d. An asterisk indicates a statistically significant difference in the means between Col and an indicated genotype, as revealed by two-tailed Student’s t -test (* P <0.05; ** P <0.01). Full size image We further examined the flowering responses in flc flm , flc flm maf2 , flc flm maf3 and flc flm maf4 mutants. Although the temperature drop-induced flowering delays in these mutants were greatly reduced, they still exhibited a weak response ( Fig. 4a ), indicating that the remaining FLC clade members in these triple mutants may act to confer the weak response. Spatial expression patterns of MAF genes overlap with those of FLC and FLM Both FLC and FLM are expressed preferentially in vasculature, shoot apices and root tips in Arabidopsis [13] , [18] . The functional redundancy among the FLC clade members prompted us to examine whether MAF2 , MAF3 and MAF4 are expressed in the same tissues as FLC and FLM . First, genomic MAF2-MAF4 fragments including a promoter region plus the entire genomic coding sequence of each gene were fused in frame with the reporter gene β-GLUCURONIDASE ( GUS ) ( Fig. 5a ). The transgenic lines expressing MAF2-GUS , MAF3-GUS or MAF4-GUS were examined by histochemical staining (for each fusion, 10–12 individual lines were checked). We found that in the seedlings MAF4 , like FLC and FLM , was preferentially expressed in vasculature such as leaf veins, shoot apices and root tips, whereas MAF2 and MAF3 were preferentially expressed in vasculature (leaf veins), in addition to a weak expression in root tips ( Fig. 5b ). Of note, FT is expressed specifically in leaf veins to promote flowering [35] ; FLC directly represses FT expression in the veins and SOC1 expression in the veins and shoot apices to inhibit flowering [13] . Taken together, these observations reveal that FLC , FLM and MAF2-MAF4 are all expressed in leaf veins, consistent with their overlapping functions in FT repression in leaf veins. 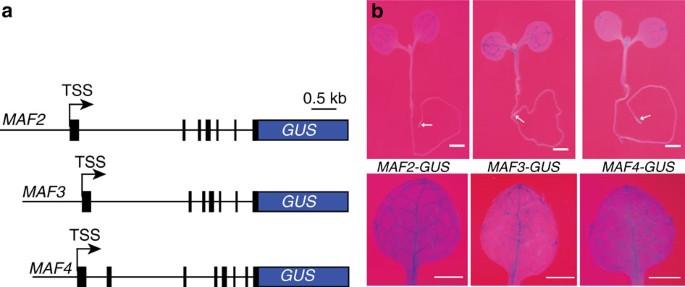Figure 5: Spatial expression patterns ofMAF2- MAF4. (a) Schematic drawings ofMAF2-,MAF3-andMAF4-GUS. Exons are represented by black, andGUSis indicated by a blue box. (b) Histochemical staining of GUS activity. Rosette leaves or 5-day-old seedlings were stained for 4 h. Scale Bar, 1.0 mm. Figure 5: Spatial expression patterns of MAF2- MAF4 . ( a ) Schematic drawings of MAF2- , MAF3- and MAF4-GUS . Exons are represented by black, and GUS is indicated by a blue box. ( b ) Histochemical staining of GUS activity. Rosette leaves or 5-day-old seedlings were stained for 4 h. Scale Bar, 1.0 mm. Full size image FLC, FLM and MAF2-MAF4 proteins form nuclear complexes Our genetic analyses have revealed complex genetic interactions among the FLC clade members: partially redundant and partially additive. We hypothesized that the FLC clade members may form MADS-domain complexes and that there may be several such complexes with different composition and partial redundancy to regulate FT expression and flowering. To test this, we first conducted yeast two-hybrid assays to check direct interactions among the FLC clade members. Direct interactions of FLC with FLM, MAF3 and MAF4, FLM with MAF2-MAF4 and MAF3 with MAF4 were observed in yeast cells ( Fig. 6a , Supplementary Fig. S9a–c ). Next, we performed biomolecular fluorescence complementation (BiFC) experiments using non-fluorescent N- and C-terminal Enhanced Yellow Fluorescent Protein (EYFP) fragments (nEYFP and cEYFP), to confirm the interactions of MAF4 with FLC and FLM, and FLM with MAF2 and MAF3 in plant cells. Indeed, when each pair of these proteins fused with nEYFP and cEYFP were transiently expressed in onion epidermal cells, YFP fluorescence was observed in the nuclei ( Fig. 6b , Supplementary Fig. S9d ), demonstrating a physical association of the two proteins in the nucleus. 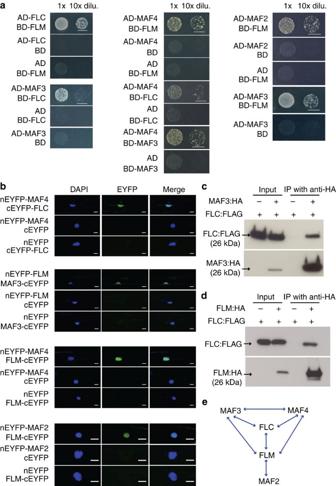Figure 6: Direct interactions among the FLC clade members. (a) Direct interactions among the FLC clade members in yeast cells. FLC, FLM and MAF2-MAF4 were fused with the GAL4-BD and/or AD domain. Yeast cells harbouring the fusion proteins, BD and/or AD, as indicated, were grown on the selective SD media lacking of Trp, Leu, His and adenine. Scale bar, 5 mm. (b) BiFC analyses of the interactions of MAF4 with FLC and FLM, and FLM with MAF2 and MAF3 in onion epidermal cells. The cells were co-transformed transiently with each pair of plasmids via biolistic gene bombardment. Yellowish-green signals resulted from the physical association of the indicated two proteins in the nuclei. Blue fluorescence from a DAPI (4′,6-diamidino-2-phenylindole) staining indicates a nucleus; scale bar, 20 μm. (c,d) Co-immunoprecipitation of FLC with MAF3 and FLM inArabidopsisseedlings. Total protein extracts from the seedlings expressing FLC:FLAG (a negative control) and F1seedlings of the doubly hemizygousFLC:FLAGandFLM:HAorFLC:FLAGandMAF3:HAwere immunoprecipitated with anti-HA agarose, followed by western blotting analysis of the precipitates with anti-FLAG. (e) Schematic representation of the direct interactions among the FLC clade members revealed in (a,b). Figure 6: Direct interactions among the FLC clade members. ( a ) Direct interactions among the FLC clade members in yeast cells. FLC, FLM and MAF2-MAF4 were fused with the GAL4-BD and/or AD domain. Yeast cells harbouring the fusion proteins, BD and/or AD, as indicated, were grown on the selective SD media lacking of Trp, Leu, His and adenine. Scale bar, 5 mm. ( b ) BiFC analyses of the interactions of MAF4 with FLC and FLM, and FLM with MAF2 and MAF3 in onion epidermal cells. The cells were co-transformed transiently with each pair of plasmids via biolistic gene bombardment. Yellowish-green signals resulted from the physical association of the indicated two proteins in the nuclei. Blue fluorescence from a DAPI (4′,6-diamidino-2-phenylindole) staining indicates a nucleus; scale bar, 20 μm. ( c , d ) Co-immunoprecipitation of FLC with MAF3 and FLM in Arabidopsis seedlings. Total protein extracts from the seedlings expressing FLC:FLAG (a negative control) and F 1 seedlings of the doubly hemizygous FLC:FLAG and FLM:HA or FLC:FLAG and MAF3:HA were immunoprecipitated with anti-HA agarose, followed by western blotting analysis of the precipitates with anti-FLAG. ( e ) Schematic representation of the direct interactions among the FLC clade members revealed in ( a , b ). Full size image We further performed in vivo co-immunoprecipitation (co-IP) experiments to determine whether MAF3 and FLM could be part of a complex with FLC in Arabidopsis . A transgenic line of Col expressing constitutively a functional FLC:FLAG [14] (note that in Col, FLC is expressed at a low level due to a non-functional fri allele), was crossed to the line expressing MAF3:HA (driven by its native promoter). We found that anti-HA (recognizing MAF3:HA) could pull down FLC:FLAG from the resulting F 1 seedlings ( Fig. 6c ), revealing that MAF3 is part of a complex with FLC. Furthermore, we crossed the FLC:FLAG line to a line expressing constitutively a functional FLM:HA fusion (see Supplementary Fig. S10a ), conducted co-IP assays with the resulting F 1 seedlings, and uncovered that FLM, like MAF3, was part of a complex with FLC ( Fig. 6d ). Taken together, our results show that the FLC clade members form nuclear MADS-domain complexes. FLC -dependent floral repression requires other FLC clade members We explored the functional dependency of FLC on other clade members. flm , maf2 and/or maf3 were introduced into FRI -Col in which the introgressed FRI activates FLC expression to inhibit flowering [36] . Given the functional redundancy of FLM with MAF2 and MAF3 , we examined the effects of flm maf2 and flm maf3 on FLC -dependent floral repression, and found that both partly suppressed the FLC -dependent late flowering of FRI -Col ( Fig. 7a ). Thus, FLM , MAF2 and MAF3 are partly required for FLC -mediated floral repression. Of note, the partial suppression in flm maf2 FRI and flm maf3 FRI may be partly attributed to that MAF2 or MAF3 is mainly expressed in leaf veins, whereas in FRI -Col, FLC is highly expressed in the shoot apex in addition to leaf veins to repress flowering [13] , [37] ; in addition, the partial functional overlapping among the FLC clade members may also contribute partly to the partial suppression. 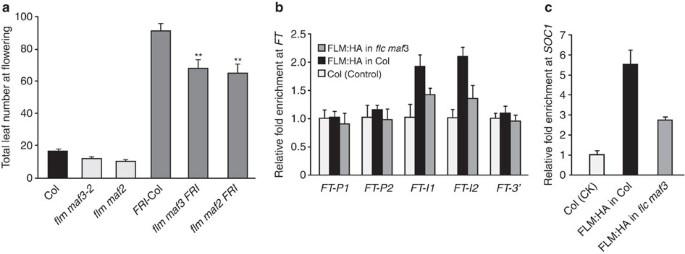Figure 7: Analysis of functional dependency ofFLCandFLMon their homologues. (a)FLC-dependent late flowering inFRI-Col requiresFLM,MAF2andMAF3. Total leaf number was scored for each line grown in LDs (12–15 plants per line). Double asterisks indicate statistically significant differences (P<0.01), revealed by two-tailed Student’st-test, in the means betweenFRI-Col andflm maf3 FRIorflm maf2 FRI. Bars indicate s.d. (b,c) ChIP analysis of FLM:HA enrichment at theFTandSOC1loci. Total chromatin was extracted from seedlings of Col (control),p35S-FLM:HA(hemizygous and functional) inFLC/− MAF3/−, andp35S-FLM:HA(hem.) inflc maf3(note that these two lines are F1progeny carrying the same transgene with nearly identical expression levels in these lines). The amounts of immunoprecipitated genomic DNA were measured by qPCR, and normalized toTUB8. The examined regions ofFTandSOC1are as described inFig. 1e, respectively. The fold enrichments of FLM:HA in each examined region in theFLM:HA-expressing lines over Col are shown. Error bars indicate s.d. of three measurements. A biological repeat of this analysis is presented asSupplementary Fig. S10b,c. Figure 7: Analysis of functional dependency of FLC and FLM on their homologues. ( a ) FLC -dependent late flowering in FRI -Col requires FLM , MAF2 and MAF3 . Total leaf number was scored for each line grown in LDs (12–15 plants per line). Double asterisks indicate statistically significant differences ( P <0.01), revealed by two-tailed Student’s t -test, in the means between FRI- Col and flm maf3 FRI or flm maf2 FRI . Bars indicate s.d. ( b , c ) ChIP analysis of FLM:HA enrichment at the FT and SOC1 loci. Total chromatin was extracted from seedlings of Col (control), p35S-FLM:HA (hemizygous and functional) in FLC/− MAF3/− , and p35S-FLM:HA (hem.) in flc maf3 (note that these two lines are F 1 progeny carrying the same transgene with nearly identical expression levels in these lines). The amounts of immunoprecipitated genomic DNA were measured by qPCR, and normalized to TUB8 . The examined regions of FT and SOC1 are as described in Fig. 1e , respectively. The fold enrichments of FLM:HA in each examined region in the FLM:HA -expressing lines over Col are shown. Error bars indicate s.d. of three measurements. A biological repeat of this analysis is presented as Supplementary Fig. S10b,c . Full size image FLM protein binds FT and SOC1 chromatin in presence of FLC clade members If FLM forms a complex with FLC and MAF3, these proteins would bind to the same region in their target gene FT and may be partly required for its binding to target chromatin. To test this, we conducted ChIPs with the WT (Col) and flc maf3 seedlings expressing a functional FLM:HA. FLM was enriched on FT chromatin, and like MAF3 and FLC FLM bound to the first and second introns, but not 5′ promoter or 3′ end of FT ( Fig. 7b , Supplementary Fig. S10b ); moreover, in the flc maf3 background the enrichments were strongly reduced compared with those in the FLM-HA-expressing WT ( Fig. 7b ), consisting with that these proteins act as part of a complex to directly repress FT expression. In addition, we found that FLM, like MAF3 and FLC, was enriched in the 5′ proximal promoter of SOC1 and that this enrichment was strongly reduced in the flc maf3 background ( Fig. 7c , Supplementary Fig. S10c ). Together, these results show that FLM binding to FT and SOC1 chromatin requires other FLC clade members, consistent with that these proteins form MADS-domain complexes to regulate flowering. In this study, we found that the FLC clade members form MADS-domain complexes to repress flowering. Environmental cues such as prolonged cold exposure, ambient temperature fluctuation and day/night cycle, and endogenous factors such as FRI and autonomous-pathway genes regulate the mRNA expression and/or protein abundance of certain FLC clade members, conceivably leading to a change in the abundance of a particular FLC–MAFs complex under a given setting. These complexes can integrate various responses to endogenous and environmental signals to modulate flowering time in Arabidopsis . We have found that the FLC clade members form nuclear complexes. Recent studies show that the MADS-domain protein SVP is in a complex with FLC for floral repression [12] , [38] . Hence, it is very likely that SVP may be part of FLC-MAFs MADS-domain complexes. Indeed, we have found that SVP can directly interact with MAF2 and MAF4 ( Supplementary Fig. S11a,b ). These findings suggest that SVP, FLC and MAFs may form higher order MADS-domain complexes. Another possibility is that SVP and the FLC clade members may form several dimeric complexes, though this is less likely because a recent study using size exclusion chromatography indicates that FLC typically exists in large protein complexes with a size more than 100 kDa [14] , much larger than the dimers of FLC with SVP or MAFs (40–50 kDa). In short, these findings collectively suggest that FLC, SVP and MAFs may form tetrameric or, less likely, dimeric complexes to regulate flowering time in Arabidopsis . MIKC c -type MADS-domain transcription factors including AGAMOUS, PISTILLATA, SEPALLATA3, APETALA1 and APETALA3 can assemble into multiple tetrameric ‘floral quartet’ complexes to control floral organ development, and several such complexes with different composition can co-exist in a cell, but may compete for DNA-binding sites such as the CArG motifs [31] . SVP, FLC and MAFs are all MIKC c -type proteins. It is likely that these proteins may form several tetrameric complexes with different composition such as FLC-SVP-MAF3-MAF4 and SVP-FLM-MAF2-MAF4. These complexes may co-exist within a cell or occur in different tissues (for example, leaf veins and the shoot apex). In this study, we have observed partial functional redundancy of FLM with FLC and MAF2-MAF4 . Given the high sequence similarity among MAF2-MAF4 (about 80% identity) [16] , functional redundancy is predicted to exist among these proteins (noteworthy, MAF2-MAF5 are arranged in a cluster that makes epistatic analyses of maf2-maf4 mutants nearly impossible [16] ). Therefore, different complexes made of FLC clade members and/or SVP (either tetrameric or dimeric) within one cell are predicted to have overlapping function in floral repression. The expression level of FT has a primary role in determining when to flower in Arabidopsis [2] , [23] . We have found that MAF3 and FLM, like FLC and SVP [12] , [13] , bind to FT chromatin (note that these four proteins are all highly enriched in the intronic region of FT ). Given the nearly identical DNA-binding domains in FLM and MAF2-MAF4, MAF2 and MAF4 are predicted to bind to FT chromatin as well. This, together with the substantial depression of FT expression in double and triple mutants of the FLC clade members, suggests that FT is a major target of the complexes composed of FLC clade members and/or SVP, particularly in the rapid-cycling accessions. Conceivably, all of these complexes could recognize and bind to the CArG motifs/variants in the FT locus (several such motifs located in the intronic and 5′ promoter regions [14] , [15] ), co-exist in companion cells of leaf veins (where FT is expressed) with different binding affinities and/or different activities for FT repression, and thus, act in partial redundancy to modulate FT expression. The mRNA expression and/or protein levels of SVP and the FLC clade members are modulated by environmental cues and endogenous factors. Vernalization represses the expression of FLC , MAF2 and FLM [16] , [39] . Growth temperature rise (for example, 23 to 27 °C) promotes alternative splicing of FLM and MAF2 pre-mRNAs, which has been postulated to cause a reduction of the isoforms encoding functional FLM and MAF2 proteins [20] . Moreover, the day/night cycles modulate diurnal abundance of SVP protein [38] . We found that the expression of MAF3, FLM and MAF2 exhibits diurnal changes as well ( Fig. 2a , Supplementary Fig. S12 ) and that MAF3 and FLM repress FT expression at the late day under inductive LDs. It has been shown that endogenous factors including FRI and gibberellins regulate FLC and SVP expression, respectively. Gibberellins repress SVP expression [12] , and in the winter annuals, the FRI protein complex activates FLC expression [5] , [6] . In short, these environmental and endogenous cues can modulate the protein levels of SVP and/or the FLC clade members, which may lead to a change in the abundance of a particular complex made of FLC, MAFs and/or SVP at a given time in the day and under a given environment, and thus confer a proper flowering time. In the rapid-cycling Arabidopsis accessions (for example, Col), FLC is repressed by the autonomous-pathway genes, whereas FLM , MAF2 , MAF3 and SVP are expressed at higher levels than FLC ( Supplementary Fig. S13 ). Thus, the MADS-domain complexes made of MAFs and/or SVP (without FLC) may be the predominant ones available for floral repression in the rapid-cycling accessions. In winter annuals, FLC expression is activated by FRI to a high level; hence, FLC-containing complexes are expected to be the major players. FLC is a potent floral repressor compared with FLM and MAF s and elevated FLC expression has a great role in floral repression. This may be attributed to that the FLC-containing complexes may possess a greater activity for gene repression, compared with the FLC-minus MADS-domain complexes, and thus strongly repress the expression of FT and SOC1 leading to late flowering and establishment of the winter-annual growth habit. Recent studies have revealed that the MADS-domain ‘floral quartet’ complexes serve as cores recruiting a few chromatin modifiers and remodelers in Arabidopsis [31] . A few chromatin modifiers such as Polycomb-repressive-complex components and histone demethylases, have been shown to directly repress FT expression [40] , [41] , [42] . A recent study suggests that FLC may exist in several complexes with a size of several hundreds of kD [14] . Hence, it is likely that the FLC-containing MADS-domain complexes may associate with these chromatin repressors and form large protein complexes at the FT locus to repress its expression. Recent genome-wide analysis of FLC-binding sites reveals that FLC directly regulates several hundred of genes [43] . Whether the FLC complexes are involved in the regulation of other FLC targets, besides FT and SOC1 , remain to be addressed in the future research. Previous studies reveal that SVP acts in the thermosensory pathway to mediate FT repression and thus flowering delay in response to a growth temperature drop (23 to 16 °C) [15] , [29] . In addition, it has been shown that FLM mediates thermosensory flowering response [20] . FLM and SVP act non-additively to repress flowering at normal growth temperature (for example, 22 °C) [19] . These observations collectively suggest that SVP and FLM may be core components in a MADS-domain complex mediating the thermosensory response. Our studies show that the flowering-delay responses in flc and maf2-maf4 mutants are partly insensitive to the growth temperature drop, similar to svp and flm mutants, though with a lesser degree. Hence, FLC and MAF2-MAF4 may form several MADS-domain complexes with the core components SVP and/or FLM, to modulate thermosensory flowering responses. In response to growth temperature rise, Arabidopsis flowers rapidly [20] , [30] . Temperature rise leads to a splicing pattern change of FLM pre-mRNAs, probably leading to a reduction in the levels of functional FLM protein [20] . It is likely that the abundance of FLM-containing MADS-domain complexes may reduce in response to temperature rise. On the other hand, temperature rise upregulates the expression of the PIF4 transcription factor that binds to FT chromatin to activate FT expression [30] . Conceivably PIF4 acts antagonistically to the complexes of SVP with FLC clade members at the FT locus to modulate its expression responding to growth temperature fluctuations. Future research is needed to understand how these two opposing activities modulate FT expression and so thermo responses of flowering. Plant materials and growth conditions The flc , flm , maf4 , maf5-1 and svp were described previously [3] , [21] , [38] , [39] . maf2 (Salk_045623), maf3-1 (Salk_022948), maf3-2 (Salk_ 070817) and maf5-2 (Salk_ 085852) alleles were isolated from the SALK collection [44] . Plants were grown in LDs (16-h light/8-h dark) or short days (8-h light/16-h dark) under cool white fluorescent light at about 22 °C except for the themosensory-flowering response assay, in which plants were grown at 16 or 23 °C in the Percival Arabidopsis growth chamber AR-41L2 with 16-h light. RNA analysis and RT-qPCR Total RNAs were extracted from aerial parts of 9 to 10-day-old seedlings grown in soils or half-MS media under LDs using Qiagen RNAeasy plus mini kit according to the manufacturer’s instructions. Subsequently, about 3.0 μg total RNAs were used as templates to synthesize cDNAs by the M-MLV reverse transcriptase (Promega). Real-time quantitative PCR was performed on an ABI Prism 7900HT sequence detection system using a SYBR Green PCR master mix. PCR was carried out as follows: 50 °C (2 min), 95 °C (10 min), followed by 40 cycles of 95 °C (15 s) and 60 °C (60 s). Each sample was quantified in triplicate, and the constitutively expressed UBQ10 and TUB2 were used as internal control genes for normalization. The primer pairs used to amply UBQ10 , TUB2 , FT , SOC1 , FD , FLM and MAF2 were described previously [45] , [46] , [47] . Primer efficiencies were determined as described by Pfaffl [48] , and calculated using the formula: E =10 −1/slope ; the efficiencies of UBQ10 , TUB2 , FT , SOC1 , FD , FLM and MAF2 primer pairs are 104%, 104%, 94%, 94%, 107%, 109% and 106%, respectively. Relative expression fold changes were determined by the comparative threshold cycle (C t ) method using the equation of 2 −ΔΔCt (both UBQ10 and TUB2 were used as the reference genes). Plasmid construction To construct MAF2-GUS , MAF3-GUS and MAF4-GUS plasmids, genomic fragments of 5.2-kb MAF2 (1.4-kb 5′ promoter plus 3.8-kb genomic coding sequence), 4.7-kb MAF3 (1.2-kb 5′ promoter plus 3.5-kb genomic coding sequence) and 4.5-kb MAF4 (0.9-kb 5′ promoter plus 3.6-kb genomic coding sequence) were inserted upstream of GUS in the pMDC162 vector [49] via gateway technology (Invitrogen), and the genomic coding sequences of MAF2, MAF3 and MAF4 were in frame with GUS . To create p35S-FLM:HA , the full-length FLM coding sequence ( AT1G77080.4 ) except the stop codon was first fused in frame with a 3xHA epitope tag, and subsequently, the fusion was inserted downstream of the 35S promoter in the pB2GW7 vector [50] via gateway technology. To create pMAF3-MAF3:HA , the 4.7-kb MAF3 genomic fragment including 1.1-kb 5′ promoter plus the entire genomic coding sequence except stop code (3.6-kb) was fused with the 3xHA tag; subsequently, the fusion was cloned into the pBGW vector [50] . Yeast two-hybrid assay The Matchmaker GAL4 Two-Hybrid System 3 (Clontech) was used for the yeast two-hybrid assays. The full-length coding sequences of FLC , FLM , MAF2 , MAF3 , MAF4 and SVP were cloned into the pGADT7 and/or pGBKT7 vectors (Clontech). Plasmids were introduced into the yeast strain AH109, and yeast cells were spotted on the SD media without leucine, tryptophan, histidine and adenine according to the manufacturer’s instructions (Clontech). BiFC assay The full-length coding sequences for FLC , FLM and MAF2 - MAF4 were fused in frame with either an N-terminal EYFP fragment in the pSAT1A-nEYFP-N1/pSAT1-nEYFPC1 vectors and/or a C-terminal EYFP fragment in the pSAT1AcEYFP-N1/pSAT1-cEYFP-C1-B vectors [51] . Plasmid pairs were introduced into onion epidermal cells by the Helium Biolistic Gene Transformation System (Bio-Rad). Within 24 h after the bombardment of a plasmid pair, the EYFP fluorescence was imaged with a Zeiss LSM 5 EXCITER upright laser scanning confocal microscopy (Zeiss). Co-immunoprecipitation Immunoprecipitation experiments were performed as described previously [45] . Briefly, total proteins were extracted from 10-day-old seedlings and immunoprecipitated with anti-HA M2 affinity gel (Sigma, Cat no. : A2220). FLC:FLAG proteins in the immunoprecipitates were detected by western blotting with anti-FLAG (Sigma, Cat no. : A8592). ChIP-quantitative PCR ChIP experiments were performed as described previously with minor modifications [52] . Briefly, total chromatin was extracted from 10-day-old seedlings and immunoprecipitated using anti-HA (Sigma, Cat no. : H6908). Quantitative PCR were performed to measure the amounts of FT , SOC1 and TUB8 (the endogenous control) fragments on an ABI Prism 7900HT sequence detection system using a SYBR Green PCR master mix. The primers used to amplify FT fragments are specified in Supplementary Table S1 . The primer pair for SOC1 were described previously [12] . The amplification efficiencies for all primer pairs were verified and the differences between the internal control TUB8 and primers for FT or SOC1 fragments are within 0.09. How to cite this article: Gu, X. et al. Arabidopsis FLC clade members form flowering-repressor complexes coordinating responses to endogenous and environmental cues. Nat. Commun. 4:1947 doi: 10.1038/ncomms2947 (2013).